The Ino80 complex mediates epigenetic centromere propagation via active removal of histone H3 The centromere is the chromosomal locus at which the kinetochore is assembled to direct chromosome segregation. The histone H3 variant, centromere protein A (CENP-A), is known to epigenetically mark active centromeres, but the mechanism by which CENP-A propagates at the centromere, replacing histone H3, remains poorly understood. Using fission yeast, here we show that the Ino80 adenosine triphosphate (ATP)-dependent chromatin-remodeling complex, which removes histone H3-containing nucleosomes from associated chromatin, promotes CENP-A Cnp1 chromatin assembly at the centromere in a redundant manner with another chromatin-remodeling factor Chd1 Hrp1 . CENP-A Cnp1 chromatin actively recruits the Ino80 complex to centromeres to elicit eviction of histone H3-containing nucleosomes. Artificial targeting of Ino80 subunits to a non-centromeric DNA sequence placed in a native centromere enhances the spreading of CENP-A Cnp1 chromatin into the non-centromeric DNA. Based on these results, we propose that CENP-A Cnp1 chromatin employs the Ino80 complex to mediate the replacement of histone H3 with CENP-A Cnp1 , and thereby reinforces itself. In most eukaryotes, centromeres are epigenetically specified by chromatin containing the centromere-specific histone H3 variant, centromere protein A (CENP-A). A model of self-propagating centromeres suggests that pre-established CENP-A chromatin at the centromeres is sufficient to direct replenishment of new CENP-A during the cell cycle [1] , [2] , [3] , [4] , [5] . At human centromeres, CENP-A replenishment occurs during G1 phase [6] and is preceded by the replication-independent loss of histone H3.3 incorporated during S phase [7] . This suggests that centromeres possess a mechanism that actively removes histone H3.3 to make room for CENP-A deposition. The fission yeast, Schizosaccharomyces pombe , has epigenetically defined “regional centromeres” whose chromatin and protein compositions are similar to those of their human counterparts [8] , [9] , [10] . In fission yeast, CENP-A Cnp1 replenishment at centromeres occurs during G2 phase in a DNA replication-independent manner [11] , and histone H3 competes with CENP-A Cnp1 for incorporation into centromeres [12] . This suggests that active removal of histone H3 may be a conserved mechanism required for CENP-A deposition at fission yeast centromeres, and makes the fission yeast an attractive genetic model for studying how histone H3 is replaced by CENP-A at regional centromeres. Adenosine triphosphate (ATP)-dependent chromatin-remodeling factors can disassemble nucleosomes and, in some cases, induce the exchange of histone variants [13] , [14] , [15] , [16] , [17] . Thus, they are good candidates to be factors through which centromeres induce the removal of histone H3. In support of this possibility, ATP-dependent chromatin-remodeling factors have been implicated in the assembly or maintenance of centromeric chromatin. In Saccharomyces cerevisiae , which has genetically defined “point centromeres” consisting of a single CENP-A Cse4 nucleosome per centromere, the Ino80 (inositol-requiring mutant 80) ATP-dependent chromatin-remodeling complex acts to maintain normal chromatin structure at centromeres [18] . However, the Ino80 complex in S. cerevisiae contributes to the integrity of pericentric chromatin rather than the assembly of CENP-A Cse4 nucleosome [18] . In humans, RSF1 (remodeling and spacing factor 1) localizes to centromeres and promotes the stable association of CENP-A with centromeres [19] . A recent study showed that RSF1 can stimulate histone exchange accompanied by CENP-A deposition when artificially targeted to ectopically inserted α-satellite DNA [20] . In addition to RSF1, the conserved ATP-dependent chromatin-remodeling factor, CHD1 (chromodomain helicase DNA binding protein 1), was found to stimulate the deposition of CENP-A Cnp1 at centromeres in human and fission yeast [21] , [22] . In these studies, however, RSF1 and CHD1 were found to be only partially involved in the deposition of CENP-A at the centromeres. This raises the possibility that other chromatin-remodeling factor(s) are also responsible for regulating CENP-A chromatin assembly at regional centromeres. Also, it remains unclear whether the critical role played by chromatin-remodeling factors at the centromeres is related to the exchange of histone H3 with CENP-A. To address these questions, here we systematically analyze the roles of the ATP-dependent chromatin-remodeling factors in the centromeric chromatin assembly of fission yeast. We find that the Ino80 complex plays an important role in CENP-A Cnp1 chromatin assembly at the fission yeast centromeres in a redundant manner with Chd1 Hrp1 , and the role of the Ino80 complex is linked to removal of histone H3-containing nucleosomes. Consistent with a direct role in CENP-A Cnp1 chromatin assembly, the Ino80 complex is associated with centromeric regions in a CENP-A Cnp1 -dependent manner and when tethered to a non-centromeric DNA inserted in an endogenous centromere promotes spreading of CENP-A Cnp1 chromatin into the non-centromeric DNA. Thus, CENP-A Cnp1 chromatin utilizes the Ino80 complex together with Chd1 Hrp1 to mediate replacement of histone H3 with CENP-A Cnp1 at regional centromeres of fission yeast. The Ino80 complex promotes CENP-A Cnp1 chromatin assembly To identify the ATP-dependent chromatin-remodeling factors involved in the replacement of histone H3 with CENP-A Cnp1 at centromeres, we first examined whether any of the fission yeast chromatin-remodeling factors could affect CENP-A Cnp1 chromatin at centromeres. The silencing of ura4 + inserted into a central core region of centromere 1 ( cnt1 : ura4 + ) was previously used to assess the integrity of CENP-A Cnp1 chromatin in fission yeast [23] , [24] . Utilizing this assay, we screened a pool of fission yeast strains carrying mutations in chromatin remodeling factors for defective central core silencing. As previously shown [21] , [25] , the loss of Chd1 Hrp1 disrupted central core silencing (Supplementary Fig. 1a, b ). In addition, we found that the loss of Ies2, a non-essential component of the Ino80 chromatin-remodeling complex, also disrupted silencing (Supplementary Fig. 1b ). Other viable mutants of the Ino80 complex, including iec1 Δ and ies6 Δ, were also defective in silencing (Fig. 1a ). Consistent with these findings, chromatin immunoprecipitation (ChIP) analyses showed that mutations of the Ino80 complex, most notably iec1 Δ and ies6 Δ, reduced the occupancy of CENP-A Cnp1 in the central core region (Fig. 1b and Supplementary Fig. 1c ). Using ChIP combined with high-throughput sequencing analysis (ChIP-Seq), we observed that the CENP-A Cnp1 levels at all centromeres were majorly reduced in ies6 Δ cells and to a smaller degree in hrp1 Δ cells (Fig. 1c and Supplementary Fig. 2 ). Defects in centromere function often increase the sensitivity of cells to microtubule-destabilizing drugs, such as thiabendazole (TBZ), and increase the rates of chromosome loss [24] , [26] . We found that iec1 Δ and ies6 Δ induce TBZ sensitivity and dramatically increase the loss of a non-essential minichromosome (Fig. 1d, e ), indicating that the impaired assembly of CENP-A Cnp1 chromatin in cells harboring defective Ino80 complex can disrupt normal centromere function. Fig. 1 Defects in the Ino80 complex impair assembly and function of centromeric chromatin. a Silencing of ura4 + inserted at centromere 1 ( cnt1 : ura4 + ) of wild-type (wt) and those harboring mutants of the Ino80 complex. The ies6 Δ, wt, and CENP-A Cnp1 mutant ( cnp1-87 ) cells were incubated for one additional day (denoted by “longer incubation”) to ensure full growth. Serial dilutions (fivefold) of cells were spotted onto non-selective (NS), uracil-depleted (−Ura), or FOA-containing (+FOA) medium at 30 °C. FOA was used to kill ura4 + -expressing cells. b Schematic of centromere 1 ( to p ), indicating the central core ( cnt ), innermost repeat ( imr ), and outer repeats ( otr/dg-dh ). The primer pairs corresponding to cnt are indicated below. ChIP analysis for CENP-A Cnp1 in the indicated cells grown at 30 °C (bottom). Fold enrichment was calculated by comparing the cnt / act1 + ratio between the IP and input DNA. Data indicate the mean±s.d. ( error bars ) of three biological replicates. c Genome browser view of centromere 1 showing the ChIP-Seq profiles of CENP-A Cnp1 . Fold enrichment represents IP relative to input. d TBZ sensitivity of cells grown with no TBZ (−TBZ) or with 10 μg ml −1 TBZ. e Minichromosome loss assay monitoring the loss of non-essential chromosome 16 (Ch16) during cell division. Cells (618–4,837) from three independent colonies for each strain were analyzed to estimate the proportion of cells in the colony containing the minichromosome (see Methods for more detail). Data indicate the mean loss rate±s.d. ( error bars ) Full size image The Ino80 complex evicts histone H3 from chromatin Next, we used ChIP-Seq to determine whether the Ino80 complex acts directly at centromeres. This analysis revealed that the Iec1 and Ies6 subunits were widely associated with central kinetochore domains (i.e., cnt and the inner parts of imr ), as well as with specific regions of pericentromeric heterochromatin ( otr ) and proximal euchromatin (Fig. 2a and Supplementary Fig. 3 ). Notably, we found that localization of the Ino80 subunits in these regions coincided with the increased levels of histone H3 in ies6 Δ and hrp1 Δ cells (Fig. 2a and Supplementary Fig. 3 ), directly implicating the Ino80 complex and Chd1 Hrp1 in the removal of histone H3-containing nucleosomes [27] . We observed that low levels of CENP-A Cnp1 incorporation were frequently observed at or near the centromere-proximal regions (pericentromeric heterochromatin and proximal euchromatin) where the Ino80 complex and Chd1 Hrp1 act to remove histone H3 (Fig. 2a and Supplementary Fig. 3 ). This suggests that the active removal of histone H3-containing nucleosomes by chromatin-remodeling factors predisposes these regions to incorporate CENP-A Cnp1 nucleosomes. The weak enrichment of CENP-A Cnp1 at these centromere-proximal regions was impaired in hrp1 Δ cells, but not in ies6 Δ cells (Fig. 2a and Supplementary Fig. 3 ). This indicates that the Ino80 complex acts primarily to remove histone H3-containing nucleosomes, which leads to the assembly of CENP-A Cnp1 in the central domain. However, unlike Chd1 Hrp1 , the Ino80 complex outside the central domain may guide only futile nucleosome exchanges, such as the reciprocal exchange of a histone H3-containing nucleosome with a CENP-A Cnp1 nucleosome, or the exchange of one histone H3-containing nucleosome with another. In contrast to ies6 Δ, the mis18-262 mutation, which disrupts kinetochore assembly [28] , was associated with reduced CENP-A Cnp1 nucleosome assembly at both central domains and centromere-proximal regions (Supplementary Fig. 4 ). This suggests that the Ino80 complex is not involved in the kinetochore-dependent deposition or maintenance of CENP-A Cnp1 . To test this further, we analyzed the effect of ies6 Δ on the centromeric localization of Scm3, a CENP-A Cnp1 -specific histone chaperone orthologous to human HJURP [29] , [30] , [31] , [32] , [33] . The association of Scm3 with centromeres is known to require various kinetochore proteins, including Sim4, Mis6, Mis16, and Mis18, but not CENP-A Cnp1 itself [ [29] . We found that binding of Scm3 to the centromere is not significantly impaired in ies6 Δ cells (Supplementary Fig. 5 ), indicating that the CENP-A Cnp1 deposition pathway is likely to be intact in ies6 Δ cells. Fig. 2 The Ino80 complex induces removal of histone H3 from associated chromatin. a ChIP-Seq profiles of CENP-A Cnp1 , Iec1-5×Flag, and Ies6-5×Flag in wt cells, and the histone H3 changes in ies6 Δ and hrp1 Δ cells relative to wt at centromere 1. The ChIP enrichments for Flag-tagged Ino80 subunits were normalized to those in mock (no tag) cells. The H3 ChIP-Seq experiments were performed and analyzed using wild-type S. cerevisiae cells as external spike-in controls (see Methods for more detail). Magnified (×10) views of CENP-A Cnp1 are shown below. The magenta and blue vertical shadings indicate the major CENP-A Cnp1 peaks in the central domain and the minor CENP-A Cnp1 peaks in the heterochromatin, respectively. b Heatmaps representing Ies6 binding in wt cells ( left ) and H3 occupancy changes in ies6 Δ cells ( right ) across all protein-coding and non-coding genes of S. pombe (from −0.5 kb of the TSS to +0.5 kb of the TES; n = 7,106). The heatmaps were sorted in descending order of Ies6 enrichment. TES, transcription termination site; TSS, transcription start site. c Average gene profiles ( n = 7,106) for Ies6 binding and histone H3 changes in ies6 Δ cells. d Venn diagram showing overlap of genes with high Ies6 binding and those with high histone H3 increases in ies6 Δ cells, as individually determined by k -means clustering ( k = 2). P -values were calculated using the hypergeometric distribution. e ChIP-Seq profiles at a representative euchromatic region for: Iec1-5×Flag; Ies6-5×Flag; histone H3 changes in ies6 Δ and hrp1 Δ cells relative to wt; and CENP-A Cnp1 in wt, ies6 Δ, and hrp1 Δ cells Full size image As in budding yeast, the Ino80 subunits of fission yeast are also associated with other genomic loci, especially near the start and end of genes [34] , [35] (Fig. 2b, c and Supplementary Fig. 6a, b ). This non-centromeric localization of the Ino80 complex allowed us to examine whether the Ino80 complex acts to remove histone H3-containing nucleosomes regardless of CENP-A Cnp1 chromatin assembly. Indeed, and consistent with the notion that the Ino80 complex plays a direct role in histone H3 removal [27] , [36] , we found that the levels of histone H3 in ies6 Δ cells were increased in regions that are normally bound by Ies6 (Fig. 2b, c ). Corroborating this, a Venn diagram analysis revealed that there is a significant overlap between genes showing high levels of Ies6 binding and those exhibiting robust increases in H3 levels in ies6 Δ cells (Fig. 2d ). We found that Chd1 Hrp1 also promotes histone H3 removal at non-centromeric regions similar to those targeted by the Ino80 complex (near the start and end of genes), but it plays a weaker role in evicting H3 from euchromatin (Fig. 2e and Supplementary Fig. 7a, b ). We also confirmed that the removal of histone H3 by the Ino80 complex at euchromatin is not tied to the assembly of CENP-A Cnp1 (Fig. 2e and Supplementary Fig. 7c ). In budding yeast, the Ino80 complex acts to remove the histone H2A variant, H2A.Z Htz1 , from chromatin [16] , [34] . Since H2A.Z Pht1 is depleted from fission yeast centromeres [37] , [38] , we questioned whether the defective CENP-A Cnp1 chromatin assembly of ies6 Δ cells could be caused by the insufficient removal of H2A.Z Pht1 , rather than H3, from the centromeres. In sharp contrast to the prominent increase in H3 occupancy seen in ies6 Δ cells, however, we found that ies6 Δ does not cause a significant increase in H2A.Z Pht1 occupancy at the centromeres (Supplementary Fig. 8a, b ). Moreover, loss of H2A.Z Pht1 did not rescue the defective central core silencing of ies2 Δ cells (Supplementary Fig. 8c ), indicating that this silencing defect is not caused by H2A.Z Pht1 . As previously reported in budding yeast [16] , [34] , we observed that H2A.Z Pht1 accumulates at both gene promoters and coding regions in ies6 Δ cells (Supplementary Fig. 8d, e ). We thus conclude that the Ino80 complex affects CENP-A Cnp1 chromatin in a manner independent of its role in restricting the localization of H2A.Z Pht1 . The action of the Ino80 complex at gene promoters prompted us to question whether the observed effect of ies6 Δ on CENP-A Cnp1 chromatin could be indirectly caused by alterations in the expression levels of specific factors that regulate CENP-A Cnp1 chromatin assembly. To exclude this possibility, we used mRNA-Seq analysis to perform gene expression profiling of ies6 Δ and wild-type (wt) cells. 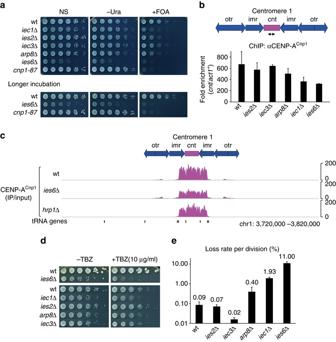Fig. 1 Defects in the Ino80 complex impair assembly and function of centromeric chromatin.aSilencing ofura4+inserted at centromere 1 (cnt1:ura4+) of wild-type (wt) and those harboring mutants of the Ino80 complex. Theies6Δ, wt, and CENP-ACnp1mutant (cnp1-87) cells were incubated for one additional day (denoted by “longer incubation”) to ensure full growth. Serial dilutions (fivefold) of cells were spotted onto non-selective (NS), uracil-depleted (−Ura), or FOA-containing (+FOA) medium at 30 °C. FOA was used to killura4+-expressing cells.bSchematic of centromere 1 (top), indicating the central core (cnt), innermost repeat (imr), and outer repeats (otr/dg-dh). The primer pairs corresponding tocntare indicated below. ChIP analysis for CENP-ACnp1in the indicated cells grown at 30 °C (bottom). Fold enrichment was calculated by comparing thecnt/act1+ratio between the IP and input DNA. Data indicate the mean±s.d. (error bars) of three biological replicates.cGenome browser view of centromere 1 showing the ChIP-Seq profiles of CENP-ACnp1. Fold enrichment represents IP relative to input.dTBZ sensitivity of cells grown with no TBZ (−TBZ) or with 10 μg ml−1TBZ.eMinichromosome loss assay monitoring the loss of non-essential chromosome 16 (Ch16) during cell division. Cells (618–4,837) from three independent colonies for each strain were analyzed to estimate the proportion of cells in the colony containing the minichromosome (see Methods for more detail). Data indicate the mean loss rate±s.d. (error bars) Consistent with the notion that the Ino80 complex plays a role in transcription, we identified hundreds of genes whose mRNA levels are significantly down- or up-regulated in ies6 Δ cells (Supplementary Table 1 ). However, among the genes whose functions are known to be important for CENP-A Cnp1 chromatin assembly, only cnp3 + , which encodes the ortholog of the CENP-A Cnp1 -binding protein, CENP-C Cnp3 , in S. pombe [39] , showed significantly reduced expression in ies6 Δ cells (Supplementary Table 1 ). A noticeable observation that we made to solve this issue was that under a suboptimal growth condition (at 25 °C in minimal EMM), ies6 Δ does not downregulate cnp3 + expression (Supplementary Fig. 9a ), but ies6 Δ cells grown under this growth condition still show a significantly reduced level of CENP-A Cnp1 at the centromere (Supplementary Fig. 9b ). Therefore, we conclude that the Ino80 complex regulates CENP-A Cnp1 chromatin regardless of its involvement in regulating cnp3 + expression. The Ino80 complex functions redundantly with Chd1 Hrp1 The weaker effect of hrp1 Δ on CENP-A Cnp1 chromatin suggests that Chd1 Hrp1 may complement the function of the Ino80 complex. We were unable to generate ies6 Δ hrp1 Δ cells, suggesting that ies6 Δ and hrp1 Δ are synthetically lethal. The ies2 Δ hrp1 Δ double-mutant cells were viable, and showed larger defects in central core silencing than those observed in each of the single mutants (Supplementary Fig. 10a ). The combination of hrp1 Δ and a mutation affecting the RSC (remodeling the structure of chromatin) chromatin-remodeling complex [40] did not produce this additive defect in silencing (Supplementary Fig. 10b, c ), nor did the RSC mutant ( rsc1 Δ) cause any silencing defect when combined with ies2 Δ (Supplementary Fig. 10d ). To further investigate the functional redundancy of Ino80 and Chd1 Hrp1 , we generated strains carrying mutations in the essential catalytic subunit, Ino80, which show a cold-sensitive central core silencing defect (see Methods for more detail). When we combined the silencing-defective ino80-11 with hrp1 Δ, we observed a cumulative loss of both silencing and cell viability (Supplementary Fig. 11a ). Consistent with this, we found that the combination of ino80-11 with hrp1 Δ produces a more prominent loss of CENP-A Cnp1 at the centromere than either of the single mutations (Supplementary Fig. 11b ). The level of histone H3 occupancy at the centromere was also increased most significantly in the double mutant ( ino80-11 hrp1 Δ) compared to the wt (Supplementary Fig. 11c ). These data indicate that Ino80 and Chd1 Hrp1 share a role in promoting the replacement of histone H3 with CENP-A Cnp1 . CENP-A Cnp1 chromatin actively recruits the Ino80 complex The association of the Ino80 complex with specific non-centromeric regions, such as gene promoters, prompted us to ask whether the centromeric localization of the Ino80 complex is mediated by CENP-A Cnp1 chromatin or by specific features of centromeric DNA sequences. To address this question, we examined whether CENP-A Cnp1 is required for the centromeric localization of the Ino80 complex. We found that in cells with defective CENP-A Cnp1 ( cnp1-1 ), the overall levels of Iec1 and Ies6 bound to the central domain ( magenta vertical shading ) were diminished and became constrained to more specific regions, including the transfer RNA genes (Fig. 3a ). Interestingly, the association of the Ino80 complex with pericentromeric heterochromatin regions ( otr ) harboring low levels of CENP-A Cnp1 ( blue vertical shading ) was completely abolished in cnp1-1 cells (Fig. 3a ). These results indicate that the widespread associations of the Ino80 complex with CENP-A Cnp1 -enriched domains occur through CENP-A Cnp1 . However, we cannot rule out the possibility that DNA sequence features may also play some role [41] . We observed that CENP-A Cnp1 , when overexpressed, co-immunoprecipitates with Ies6, which raises the possibility that CENP-A Cnp1 may have an interaction with the Ino80 complex (Supplementary Fig. 12 ). To further evaluate the significance of CENP-A Cnp1 chromatin or DNA sequence cues in the centromeric localization of the Ino80 complex, we utilized a neocentromere strain that lacks the endogenous centromere of chromosome 1 and carries an ectopic centromere assembled at a non-centromeric region near the right telomere of chromosome 1 ( tel1R-neocen ) without any DNA sequence change [42] (Fig. 3b ). We found that Ies6 is widely associated with the tel1R-neocen locus in the neocentromere strain but not in the wt strain (Fig. 3c ). Thus, CENP-A Cnp1 chromatin, not the DNA sequence, majorly contributes to localizing the Ino80 complex to the neocentromere. Fig. 3 The Ino80 complex is recruited to centromeres through CENP-A Cnp1 chromatin. a Magnified (×10) views of CENP-A Cnp1 in wt cells and ChIP-Seq profiles of Ies6-5×Flag and Iec1-5×Flag in wt and cnp1-1 cells at centromere 1. For Flag ChIP-Seq, wt and cnp1-1 cells were incubated at 36 °C (restrictive temperature for cnp1-1 ) for 3 h after being grown at 25 °C (permissive temperature for cnp1-1 ). The magenta and blue vertical shadings indicate the major CENP-A Cnp1 peaks in the central domain and the minor CENP-A Cnp1 peaks in the heterochromatin, respectively. b A schematic showing the positions of active centromeres ( white circles ) in chromosome 1 of the wt and neocentromere (neocen) strains. The neocentromere strain carries a neocentromere ( tel1R-neocen ) assembled at a subtelomeric region, but lacks the endogenous centromere 1 ( cen1 Δ; white box ). c Genome browser view of the tel1R-neocen locus showing the ChIP-Seq profiles of CENP-A Cnp1 , histone H3, and Ies6-5×Flag in the wt and neocentromere strains. The blue vertical shadings indicate the major CENP-A Cnp1 peaks in the neocentromere Full size image Tethered Ino80 subunits promote spreading of CENP-A Cnp1 A large non-centromeric DNA placed in an endogenous centromere was previously shown to act as a poor substrate for the spreading of CENP-A Cnp1 chromatin [43] . We used this to more directly address the function of the Ino80 complex in CENP-A Cnp1 chromatin assembly. We tethered a TetR-2×Flag-Iec1 (TetR-Iec1) fusion to tetO sites in a 4.5 kb non-centromeric DNA ( bighyg ) sequence inserted at centromere 1, and examined whether tethered TetR-Iec1 alters CENP-A Cnp1 chromatin assembly at bighyg (Fig. 4a ). We used TetR-2×Flag alone (TetR) and TetR-Iec1 released from bighyg by anhydrotetracycline (AHT) treatment as negative controls. We used ChIP analysis to confirm that TetR and TetR-Iec1 were enriched at tetO insertions and that TetR-Iec1 was released after the addition of AHT (Fig. 4b ). A subsequent ChIP-Seq analysis showed that tethered TetR-Iec1 triggered the spread of CENP-A Cnp1 chromatin into bighyg concurrent with a decline in histone H3 occupancy (Fig. 4c , compare TetR-Iec1 with TetR or TetR-Iec1+AHT). Tethering of TetR-Iec1 to more central regions of bighyg did not cause such a robust increase in CENP-A Cnp1 chromatin assembly ( gray vertical shadings in Fig. 4c ). However, TetR-Iec1 tethered to these regions causes a more notable local histone H3 depletion relative to surrounding regions than did tethered TetR ( gray vertical shadings in Fig. 4c ), which is consistent with the notion that TetR-Iec1 induces the removal of histone H3-containing nucleosomes around the tethered sites. To determine whether the effect of tethered TetR-Iec1 reflects the underlying catalytic activity of the Ino80 complex, we ectopically expressed TetR-Ino80 or TetR-Ino80 K873A , which has a mutation in its conserved ATP-binding pocket [44] , [45] . We observed similar enrichments for TetR, TetR-Ino80, and TetR-Ino80 K873A at tetO insertions, and TetR-Ino80 was successfully released after the addition of AHT (Fig. 4d ). However, tethered TetR-Ino80, but not TetR-Ino80 K873A , caused the spreading of CENP-A Cnp1 chromatin into bighyg (Fig. 4e , compare TetR-Ino80 and TetR-Ino80 K873A at p1, p2, and p10), clearly implicating the ATPase activity of Ino80 in CENP-A Cnp1 chromatin assembly. Moreover, we found that tethered Ino80 subunits exert a stronger effect on CENP-A Cnp1 assembly when placed closer to the native centromere (Fig. 4c–e ). This supports that the Ino80 complex needs to be in a kinetochore context to stimulate CENP-A Cnp1 chromatin assembly, which is consistent with the observation that CENP-A Cnp1 does not accumulate at non-centromeric regions where the Ino80 complex acts to remove histone H3 (Fig. 2e and Supplementary Fig. 7c ). Fig. 4 Tethered Ino80 subunits enhance spreading of CENP-A Cnp1 chromatin into a non-centromeric DNA. a A schematic of cnt1 : bighyg showing the positions of the tet operators ( tetO ), the TetR fusion proteins (or TetR alone) in bighyg . The bighyg DNA consists of ura4 + , arg3 + coding sequence ( arg3-cds ), and the hygromycin-resistance gene ( hphMX6 ). The utilized primers pairs are indicated below. b ChIP analysis for Flag-tagged TetR, TetR-Iec1, and TetR-Iec1 in cells treated with AHT (TetR-Iec1+AHT), as assessed using the indicated primers. TetR-Iec1 binding was significantly reduced after the addition of AHT, as determined by Student’s t -tests (* P ≤ 0.05, ** P ≤ 0.01, and *** P ≤ 0.001). c Genome browser view of bighyg ( top ) and centromere 1 ( bottom ) showing the ChIP-Seq profiles of CENP-A Cnp1 ( magenta ) and histone H3 ( blue ) in TetR-expressing cells, TetR-Iec1-expressing cells, and TetR-Iec1-expressing cells treated with AHT (TetR-Iec1+AHT). Gray vertical shadings indicate ~400 bp regions encompassing tetO inserted in the central part of bighyg . d ChIP analysis for Flag-tagged TetR, TetR-Ino80, TetR-Ino80 K873A , and TetR-Ino80 in cells treated with AHT (TetR-Ino80+AHT), as assessed using the indicated primers. e ChIP analysis for CENP-A Cnp1 in cells expressing Flag-tagged TetR, TetR-Ino80, and TetR-Ino80 K873A , and in TetR-Ino80-expressing cells treated with AHT (TetR-Ino80+AHT), as assessed using the indicated primers. Error bars in all ChIP data indicate the ±s.d. for the biological replicates Full size image This study shows that the Ino80 complex is a critical chromatin-remodeling factor required for CENP-A Cnp1 chromatin assembly at the centromeres of fission yeast. Chd1 Hrp1 , which was previously implicated in CENP-A Cnp1 chromatin assembly [21] , plays a redundant role with the Ino80 complex. Our findings in fission yeast may explain the discrepancy between human and Drosophila regarding the involvement of CHD1 in CENP-A chromatin assembly [22] , [46] , as the function of CHD1 could be easily concealed by the redundant function of other chromatin-remodeling factors such as the Ino80 complex. Our conclusion that CENP-A Cnp1 chromatin rather than specific DNA sequence is the major determinant for centromeric localization of the Ino80 complex is supported by two main observations. First, the binding of Ino80 subunits is detected across the CENP-A Cnp1 chromatin domains, and this widespread association is largely dependent on CENP-A Cnp1 (Fig. 3a ). Second, Ies6 associates with the site of neocentromere formation only when the neocentromere is activated and CENP-A Cnp1 chromatin is assembled on the DNA (Fig. 3c ). Previous studies showed that the Ino80 complex in budding yeast also associates with the centromeres [47] and promotes pericentric chromatin integrity and centromere function [18] , but does not affect the assembly of CENP-A Cse4 nucleosomes at the centromeres [18] . A recent study uncovered a rather unexpected role for the budding yeast Ino80 complex in promoting the ectopic deposition of CENP-A Cse4 at gene promoters [48] . We speculate that the requirement for the Ino80 complex in the assembly of CENP-A nucleosomes at the centromeres was lost in budding yeast during the evolutionary transition from regional to point centromeres [49] . In contrast, the connection of the Ino80 complex with centromeres [18] and CENP-A [48] was retained, allowing the Ino80 complex to exhibit divergent roles in budding yeast. The roles of the Ino80 complex in CENP-A chromatin assembly at regional versus point centromeres should be examined in the future to test this hypothesis. As reported in budding yeast [16] , [34] , we herein show that the fission yeast Ino80 complex plays a prominent role in removing histone H2A.Z Pht1 from chromatin (Supplementary Fig. 8d, e ). However, we found that H2A.Z Pht1 does not significantly accumulate at the centromeres in ies6 Δ cells (Supplementary Fig. 8a, b ) and the defective central core silencing in ies2 Δ cells is not rescued by the elimination of histone H2A.Z Pht1 (Supplementary Fig. 8c ). These results indicate that the major function of the Ino80 complex in the assembly of CENP-A Cnp1 chromatin at the centromeres is not likely to be the removal of histone H2A.Z Pht1 . Instead, our analysis revealed that the localization of the Ino80 complex was tightly correlated with its role in histone H3 eviction rather than CENP-A Cnp1 deposition (Fig. 2 ). Our findings thus support a model in which the Ino80 complex mainly acts at the centromeres to remove histone H3-containing nucleosomes as a prerequisite for CENP-A Cnp1 deposition. We note that the Ino80 complex was also shown to induce full nucleosome turnover in budding yeast [34] . Kinetochore proteins, such as CENP-C Cnp3 , may stabilize CENP-A Cnp1 nucleosomes at centromeres [50] , thereby generating a chromatin context in which the Ino80 complex selectively evicts histone H3-containing nucleosomes. Extending our model, a recent study showed that the chromatin-remodeling factor, RSF1, can stimulate histone H3.3 exchange as well as CENP-A deposition in humans [20] . Based on the present and prior findings, we envision that the exchange of histone H3-containing nucleosomes with CENP-A nucleosomes by centromere-targeted chromatin-remodeling factors could be a conserved theme underpinning the epigenetic propagation of CENP-A chromatin at regional centromeres. Strains, drugs and standard techniques Standard genetic and molecular techniques were used. YES (Yeast Extract with Supplements) was used as a rich medium and PMG (Pombe Minimal Glutamate) or EMM (Edinburgh Minimal Medium) was used as a minimal medium. For the selective and non-selective media in the silencing assays, we used PMG supplemented with amino acids. For 5-fluoroorotic acid (FOA) selection, we added FOA (final concentration 1 g l −1 ) to PMG media. Where indicated, we added TBZ (final concentration 10 μg ml −1 ; Sigma) dissolved in dimethyl sulfoxide to the YES plates and AHT (final concentration 10 μM; Sigma) dissolved in DMSO to the YES or PMG media. We incubated all fission yeast cells at 30 °C unless otherwise indicated. We used PCR-based gene targeting or genetic crosses followed by random spore analysis to create the deletion and Flag-tagged strains. We were able to infer the synthetic lethality of ies6 Δ hrp1 Δ by crossing ies6 Δ and hrp1 Δ and performing a random spore analysis; we were unable to find any ies6 Δ:: natMX6 hrp1 Δ:: kanMX6 ( nat R kan R ) spores despite selecting over 300 ies6 Δ:: natMX6 ( nat R ) spores. 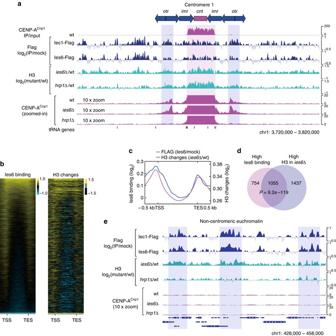Fig. 2 The Ino80 complex induces removal of histone H3 from associated chromatin.aChIP-Seq profiles of CENP-ACnp1, Iec1-5×Flag, and Ies6-5×Flag in wt cells, and the histone H3 changes inies6Δ andhrp1Δ cells relative to wt at centromere 1. The ChIP enrichments for Flag-tagged Ino80 subunits were normalized to those in mock (no tag) cells. The H3 ChIP-Seq experiments were performed and analyzed using wild-typeS. cerevisiaecells as external spike-in controls (see Methods for more detail). Magnified (×10) views of CENP-ACnp1are shown below. Themagentaandblue vertical shadingsindicate the major CENP-ACnp1peaks in the central domain and the minor CENP-ACnp1peaks in the heterochromatin, respectively.bHeatmaps representing Ies6 binding in wt cells (left) and H3 occupancy changes inies6Δ cells (right) across all protein-coding and non-coding genes ofS. pombe(from −0.5 kb of the TSS to +0.5 kb of the TES;n= 7,106). The heatmaps were sorted in descending order of Ies6 enrichment. TES, transcription termination site; TSS, transcription start site.cAverage gene profiles (n= 7,106) for Ies6 binding and histone H3 changes inies6Δ cells.dVenn diagram showing overlap of genes with high Ies6 binding and those with high histone H3 increases inies6Δ cells, as individually determined byk-means clustering (k= 2).P-values were calculated using the hypergeometric distribution.eChIP-Seq profiles at a representative euchromatic region for: Iec1-5×Flag; Ies6-5×Flag; histone H3 changes inies6Δ andhrp1Δ cells relative to wt; and CENP-ACnp1in wt,ies6Δ, andhrp1Δ cells For more details regarding the yeast strains used in each experiment, see Supplementary Table 2 . ChIP-Seq and data analysis Cells were fixed with 1% formaldehyde for 10 min (for cells grown at 36 °C), 15 min (for cells grown at 30 °C), or 40 min (for cells grown at 20 °C). ChIP-Seq required more cells than conventional ChIP, as we needed to ensure that there was sufficient immunoprecipitated DNA for high-throughput sequencing. We used 1.6 × 10 9 , 4 × 10 8 , and 2.4–3.2 × 10 9 cells for the CENP-A Cnp1 ChIP, H3 ChIP, and Flag ChIP experiments, respectively, increasing the amount of lysis buffers and antibodies accordingly. For the CENP-A Cnp1 and H3 ChIP-Seq, we used 70 µl of in-house rabbit anti-CENP-A Cnp1 antiserum and 15 µl of in-house rabbit anti-H3 antiserum, respectively. For the Flag ChIP-Seq experiments, we used 10 µl of anti-Flag M2 antibody (1 mg ml −1 , mouse monoclonal, F1804; Sigma) and included equal numbers of wt cells (lacking any tag) in parallel as controls. We performed the ChIP experiments for CENP-A Cnp1 and H3 with only minor modifications to conventional ChIP protocols. We prepared the cell extracts by disrupting the cells in lysis buffer (50 mM HEPES-KOH, pH 7.5, 140 mM NaCl, 1 mM EDTA, 1% Triton X-100, 0.1% sodium deoxycholate) using a standard bead-beating protocol. Following immunoprecipitation (IP), we washed the DNA-bound protein Aagarose beads and eluted the DNA in IP columns (SigmaPrep spin columns, Sigma) instead of microfuge tubes. As the external spike-in control for the H3 ChIP-Seq experiments, formaldehyde-fixed wild-type S. cerevisiae (W303a) cells were added to the S. pombe cells at a 1:8 ratio before cell disruption. For the Flag ChIP experiments, we used a modified lysis buffer (50 mM Tris-HCl, pH 7.5, 150 mM NaCl, 1 mM EDTA, 1% Triton X-100) and Tris-buffered saline (TBS) (20 mM Tris-HCl, pH 7.5, 150 mM NaCl)-based wash buffers (TBS and TBS with 0.05% Tween-20) to avoid denaturation of the M2 antibody by sodium deoxycholate. As the external spike-in control for the H2A.Z Pht1 -5×Flag ChIP-Seq experiments, formaldehyde-fixed S. cerevisiae cells expressing Sua7-5×Flag were added to S. pombe cells at a 1:9 ratio before cell disruption. We recovered the de-crosslinked DNA using a Qiagen PCR purification kit. We constructed the ChIP-Seq libraries with 5 to 10 ng of input DNA or 1 to 10 ng of immunoprecipitated DNA, using a ChIP-Seq kit (NEXTflexChIP-Seq kit, Bioo Scientific) according to the manufacturer’s protocol. For multiplexed libraries, we sequenced 50 nt single-end reads on an Illumina HiSeq 2500 (Theragen and Macrogen). After removing the adapter sequences, we aligned the processed reads to the S. pombe ASM294v2 genome assembly using Novoalign. We randomly assigned single locations to reads that mapped to multiple locations. For reads obtained from duplicate samples, we confirmed their experimental reproducibility using the bamCorrelate tool from the deepTools package [51] . For quantitative analysis of the data obtained from the H3 and H2A.Z Pht1 ChIP-Seq experiments, we calculated the IP/input ratio for each ChIP normalized to that of the spike-in control, which in principle should be constant in all ChIP samples. The normalized ratio of IP/input (E IP ) was derived as: E IP =(read count of IP mapped to S. pombe genome/read count of input mapped to S. pombe genome)/(read count of IP mapped to S. cerevisiae genome/read count of input mapped to S. cerevisiae genome). We computed the fold change of IP versus the input using the deepToolsbamCompare tool. The normalization factor ( N ) for the IP/input in each ChIP-Seq experiment was calculated as: N ×read count of IP/read count of input=E IP :1. When we directly computed the fold change of IP in the mutant versus wild type, the normalization factor ( N ) for IP mutant /IP wt was calculated as: N ×read count of IP mutant /read count of IP wt =E IP of mutant/E IP of wt. The normalization of ChIP-Seq for CENP-A Cnp1 , Iec1-5×Flag and Ies6-5×Flag was performed using the signal extraction scaling method. For visualization of the normalized data, we used the integrative genome viewer. We used the deepTools computeMatrix tool to perform an average gene (metagene) analysis and the profiler tool from deepTools to visualize the average gene profiles. We generated heatmaps using the deepToolsHeatmapper. We performed all further downstream bioinformatic analyses of the ChIP-Seq data using the R software package. ChIP analysis We performed the Fast ChIP protocol [52] using 20 µl of anti-CENP-A Cnp1 antibody (rabbit polyclonal; in-house), 8 µl of anti-H3 antibody (rabbit polyclonal; in-house), 2 µl of anti-Flag M2 antibody (1 mg ml −1 , mouse monoclonal, F1804; Sigma), and 2 µl of anti-GFP tag antibody (2 mg ml −1 , rabbit polyclonal, A-11122; Thermo Fisher). We used the Bio-Rad CFX96 system to analyze the input or IP DNA by quantitative PCR. 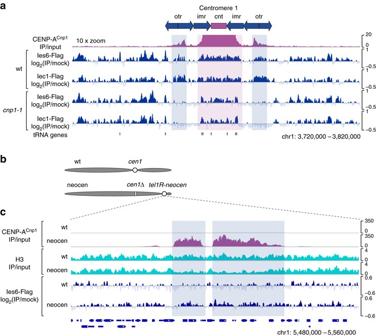Fig. 3 The Ino80 complex is recruited to centromeres through CENP-ACnp1chromatin.aMagnified (×10) views of CENP-ACnp1in wt cells and ChIP-Seq profiles of Ies6-5×Flag and Iec1-5×Flag in wt andcnp1-1cells at centromere 1. For Flag ChIP-Seq, wt andcnp1-1cells were incubated at 36 °C (restrictive temperature forcnp1-1) for 3 h after being grown at 25 °C (permissive temperature forcnp1-1). Themagentaandblue vertical shadingsindicate the major CENP-ACnp1peaks in the central domain and the minor CENP-ACnp1peaks in the heterochromatin, respectively.bA schematic showing the positions of active centromeres (white circles) in chromosome 1 of the wt and neocentromere (neocen) strains. The neocentromere strain carries a neocentromere (tel1R-neocen) assembled at a subtelomeric region, but lacks the endogenous centromere 1 (cen1Δ;white box).cGenome browser view of thetel1R-neocenlocus showing the ChIP-Seq profiles of CENP-ACnp1, histone H3, and Ies6-5×Flag in the wt and neocentromere strains. Theblue vertical shadingsindicate the major CENP-ACnp1peaks in the neocentromere 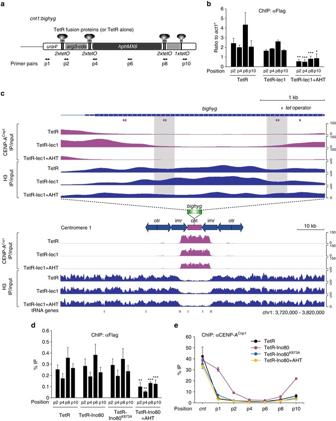Fig. 4 Tethered Ino80 subunits enhance spreading of CENP-ACnp1chromatin into a non-centromeric DNA.aA schematic ofcnt1:bighygshowing the positions of thetetoperators (tetO), the TetR fusion proteins (or TetR alone) inbighyg. ThebighygDNA consists ofura4+,arg3+coding sequence (arg3-cds), and the hygromycin-resistance gene (hphMX6). The utilized primers pairs are indicated below.bChIP analysis for Flag-tagged TetR, TetR-Iec1, and TetR-Iec1 in cells treated with AHT (TetR-Iec1+AHT), as assessed using the indicated primers. TetR-Iec1 binding was significantly reduced after the addition of AHT, as determined by Student’st-tests (*P≤ 0.05, **P ≤0.01, and ***P≤ 0.001).cGenome browser view ofbighyg(top) and centromere 1 (bottom) showing the ChIP-Seq profiles of CENP-ACnp1(magenta) and histone H3 (blue) in TetR-expressing cells, TetR-Iec1-expressing cells, and TetR-Iec1-expressing cells treated with AHT (TetR-Iec1+AHT).Gray vertical shadingsindicate ~400 bp regions encompassingtetOinserted in the central part ofbighyg.dChIP analysis for Flag-tagged TetR, TetR-Ino80, TetR-Ino80K873A, and TetR-Ino80 in cells treated with AHT (TetR-Ino80+AHT), as assessed using the indicated primers.eChIP analysis for CENP-ACnp1in cells expressing Flag-tagged TetR, TetR-Ino80, and TetR-Ino80K873A, and in TetR-Ino80-expressing cells treated with AHT (TetR-Ino80+AHT), as assessed using the indicated primers.Error barsin all ChIP data indicate the ±s.d. for the biological replicates See Supplementary Table 3 for the primer sequences. mRNA-Seq analysis We extracted total RNAs and isolated mRNAs from wt and ies6 Δ cells using poly(A)beads (NEXTflex). The stranded libraries were generated from biological replicates of each strain using NEXTflex Rapid Directional RNA-Seq Kit according to the manufacturer’s manual and sequenced as single end. The sequence reads were aligned using STAR aligner [53] . Cufflinks tools were used to assemble the transcripts, to calculate their abundance in FPKM, and to determine list of genes that are differentially expressed in ies6 Δ cells compared to wt. Genes whose expressions were increased or decreased more than twofold in ies6 Δ cells relative to wt with q -value (false discovery rate-adjusted p -value) of ˂0.05 were defined as significantly upregulated or downregulated genes, respectively (Supplementary Table 1 ). Generation of silencing-defective alleles of ino80 + To identify mutant alleles of ino80 + , we used a Gene Morph II random mutagenesis kit (Stratagene) to mutagenize a DNA fragment containing the terminal 1.4 kb of the ino80 + open reading frame (ORF), which covered a significant portion of the catalytic domain. We then used fusion PCR to fuse the mutagenized fragments to a kan R marker gene and sequences downstream of the ino80 + ORF. We selected transformants on G418-containing plates by screening for slow growth at 35.5 °C. Then, we further screened these mutants for defective silencing of cnt1:ura4 + at different temperatures (25, 30, 32.5, 35.5 °C). This technique allowed us to isolate several cold-sensitive silencing-defective mutant alleles, including ino80-11 . We identified the respective causative mutations in selected each strain using standard Sanger sequencing. Minichromosome loss assay We used genetic crossing to introduce a non-essential minichromosome (chromosome 16 (Ch16)). Ch16 bears the S. cerevisiae LEU2 gene, which allows it to complement leu1-32 . We cultured wt and mutant cells containing Ch16 in minimal medium lacking leucine (PMG-Leu) to maintain the minichromosome. We plated these cells on non-selective (YES) plates with or without allowing them to divide 10 to 12 times in non-selective medium (YES). We then replica-plated the resulting colonies onto selective medium lacking leucine (PMG-Leu) and counted those that could and could not grow on selective medium (PMG-Leu). We calculated the rate of minichromosome loss using the following formula: loss rate per division (%)=100 × (1−( F / I ) 1/ N ), where F is the final percentage of minichromosome-containing cells, I is the initial percentage of minichromosome-containing cells, and N is the number of generations [54] . We tested three independent colonies for each strain. Data are presented as the mean loss rate±s.d. (error bars). Co-immunoprecipitation Cell pellets from log-phase cultures were resuspended in NP40 lysis buffer (1% NP40, 200 mM NaCl, 2 mM EDTA, 6 mM Na 2 HPO4, 4 mM NaH 2 PO 4 , 2 mM PMSF, protease inhibitors) and lysed by bead-beating. Extracts were immunoprecipitated with 25 µl anti-Flag (M2)-agarose (Sigma). Immunoprecipitates were subjected to western blotting for the presence of Ies6-5×Flag or CENP-A Cnp1 using horseradish peroxidase-conjugated anti-Flag (M2) antibody (1:5,000, A8592; Sigma) or affinity-purified anti-CENP-A Cnp1 antibody (1:1,000; in-house), respectively. Generation of tethering strains We generated the cnt1 : bighyg strain based on the cnt1 : ura4 + strain, which contains ura4 + at the Nco I site of the central core region in centromere 1 [23] . First, we used PCR to attach 2× tetO or 1× tetO to each end of a 1 kb DNA fragment derived from the internal coding region of arg3 + . We then integrated the resulting PCR fragments into the middle of ura4 + and integrated the hygromycin-resistance gene ( hphMX6 ), which is flanked by 2× tetO , into the center of the arg3 + insertion. Finally, we deleted the endogenous ura4 + and arg3 + genes of the resulting cnt1 : bighyg strain. The ura4 + terminator sequence at the end of cnt1:bighyg was excluded from the analysis because it is also present at the end of the endogenous ura4 + locus. We generated the TetR-2×Flag-Iec1 fusion strain by replacing the start codon (ATG) of the endogenous iec1 + gene with a DNA fragment encoding TetR-2×Flag. We generated the TetR-2×Flag strain without the Iec1 fusion by fusing the iec1 + promoter and the TetR-2×Flag sequence and integrating them into an ectopic ura4 + locus to replace the promoter and coding region of ura4 + . For the Ino80-tethering experiments, we replaced the promoter and coding region of ura4 + with the thiamine-repressible nmt81 promoter and a DNA sequence encoding TetR-2×Flag-Ino80, TetR-2×Flag-Ino80 K873A , or TetR-2×Flag. We induced expression of the fusion proteins by growing the strains in PMG medium lacking thiamine. We generated the TetR fusion gene-containing strains and cnt1 : bighyg by genetic crosses and verified them using diagnostic PCR. Data availability The raw and processed sequencing data from this publication have been submitted to the NCBI Gene Expression Omnibus (GEO; http://www.ncbi.nlm.nih.gov/geo/ ) under accession number GSE99589. The authors declare that all the data supporting the findings of this study are available within the article and its Supplementary Information files and from the corresponding author on reasonable request.